LUX ARRHYTHMO mediates crosstalk between the circadian clock and defense in Arabidopsis The circadian clock is known to regulate plant innate immunity but the underlying mechanism of this regulation remains largely unclear. We show here that mutations in the core clock component LUX ARRHYTHMO (LUX) disrupt circadian regulation of stomata under free running and Pseudomonas syringae challenge conditions as well as defense signaling mediated by SA and JA, leading to compromised disease resistance. RNA-seq analysis reveals that both clock- and defense-related genes are regulated by LUX. LUX binds to clock gene promoters that have not been shown before, expanding the clock gene networks that require LUX function. LUX also binds to the promoters of EDS1 and JAZ5 , likely acting through these genes to affect SA- and JA-signaling. We further show that JA signaling reciprocally affects clock activity. Thus, our data support crosstalk between the circadian clock and plant innate immunity and imply an important role of LUX in this process. In response to various pathogens and pests, plants have evolved sophisticated defense mechanisms to recognize and fight these invaders. One such mechanism uses the internal time measuring machinery, the circadian clock, to modulate defense responses in anticipation of pathogens and pests at the time of day when they are likely to be encountered as well as during an actual attack [1] . The circadian clock is known to have a profound influence on plant growth, development, and responses to environmental cues [2] , [3] , [4] , although the mechanisms by which the circadian clock regulates plant defense are only beginning to be elucidated. Although the molecular composition of the circadian clock differs greatly between plants and other organisms, the basic principle of clock function, which is the ability to self-sustain an approximately 24-h cycle, is conserved. Like in other organisms, the circadian clock in plants consists of core clock components, which form complicated interlocking transcription–translation feedback loops (TTFLs) that are subject to both transcriptional and posttranscriptional regulation [2] , [3] , [4] . Core clock genes are expressed at different times of a day and can affect the expression and/or activities of each other as well as of genes acting in output pathways. The concerted function of these clock genes calibrates the circadian clock and keeps timing in a precise, self-sustaining manner. For instance, the two homologous Myb transcription factors, CIRCADIAN CLOCK-ASSOCIATED 1 ( CCA1 ) and LATE ELONGATED HYPOCOTYL ( LHY ), are expressed in the morning (morning-phased) and contribute to multiple clock TTFLs through a direct regulation of several other core clock genes and themselves. CCA1 and LHY also directly regulate the expression of many clock output genes [5] . One target of the CCA1 protein is the evening-phased core clock gene LUX ARRHYTHMO ( LUX ), also known as PHYTOCLOCK1 , which encodes a GARP transcription factor essential for circadian rhythmicity [6] , [7] . Expression of LUX is also affected by several other clock proteins, including TIMING OF CAB EXPRESSION 1 (TOC1), REVEILLE 8 (RVE8), PSEUDO-RESPONSE REGULATOR 5 (PRR5), and PRR7 [8] , [9] , [10] , [11] . In turn, LUX binds directly to the conserved LUX-binding site (LBS) in the promoters of several clock genes, including GIGANTEA ( GI ), NIGHT LIGHT-INDUCIBLE AND CLOCK-REGULATED GENE 1 ( LNK1 ), PRR7 , PRR9 , and LUX itself, to regulate their expression [7] , [12] . Thus, like CCA1 and LHY , LUX is involved in multiple clock TTFLs. LUX, at least in part, functions through interactions with other proteins. LUX or its close homolog, BROTHER OF LUX ARRHYTHMO (BOA), forms the evening complex (EC) with two evening-phased proteins, EARLY FLOWERING 3 (ELF3) and ELF4 [13] , [14] . The EC affects many aspects of plant development and physiology, including growth, flowering, and cold response, as clock outputs [15] . Recent studies have demonstrated a critical role of the circadian clock in plant defense against pathogens and pests. Disruption of certain clock genes leads to reduced resistance against bacteria, oomycete, and/or fungal pathogens [1] . Arrhythmicity caused by misexpressing LUX or CCA1 compromises insect resistance [16] . The temporal control of defense by the circadian clock manifests in the rhythmic changes of defense-related molecules, reflecting the role of the circadian clock in anticipating likely attacks from pathogens and pests. For instance, in the absence of pathogens and pests, expression of many defense-related genes and production of defense signaling molecules, such as salicylic acid (SA), jasmonic acid (JA), and reactive oxygen species (ROS), oscillate with varying peaks during the day [16] , [17] , [18] , [19] . However, in the presence of pathogens and pests, plants activate acute defense responses, including drastic increases in SA and other defense compounds and reprogramming of defense-related genes. Most of these acute responses lose the rhythmic signature observed under the unchallenged condition. For instance, while the levels of SA oscillate daily in unchallenged plants [16] , [17] , timely accumulation of SA in high abundance in the local infected region dictates the outcome of plant response to some pathogens [20] , [21] . Genes affecting such acute SA accumulation are important for plant defense [22] , [23] , [24] , although no clock genes have yet been reported to play such a role in SA regulation. Thus how the circadian clock gates acute defense responses in the presence of pathogens and pests remains largely unknown. In order to identify circadian clock genes that contribute to SA regulation, we conducted a genetic analysis with a unique Arabidopsis mutant, acd6-1 , which exhibits constitutively high levels of defense that are inversely correlated with the size of the plant [25] , [26] . This feature of acd6-1 has proven useful in gauging the effects of potential mutations on defense [21] , [22] , [27] , [28] , [29] , [30] , [31] . We report here that lux-1 , a nonsense mutation in the early coding region of the LUX gene [6] , suppresses acd6-1 -conferred dwarfism and high SA defense phenotypes. We confirmed the SA regulatory role of LUX with Pseudomonas syringae infection and further discovered a role of LUX in regulating JA signaling. This function of LUX arises, at least in part, through a direct control of the key SA and JA signaling genes, ENHANCED DISEASE SUSCEPTIBILITY ( EDS1 ) [27] , [32] and JASMONATE ZIM-DOMAIN 5 ( JAZ5 ) [33] , [34] , respectively. LUX also affects temporal stomatal opening and closure under free running and acute pathogen challenging conditions. Consistent with the multiple functions of LUX in defense regulation, lux-1 is compromised in resistance to a broad spectrum of pathogens and pests. RNA-seq analysis followed by chromatin immunoprecipitation (ChIP) experiments supports a central role of LUX in clock and defense regulation. In addition, we show that activation of JA signaling affects LUX expression and reciprocally regulates clock activity. Together, our data reveal an important role of LUX mediating the crosstalk between the circadian clock and plant innate immunity. LUX regulates SA-mediated defense In order to identify circadian clock genes that gate plant defense, especially SA-mediated defense, we introduced several clock mutations into acd6-1 , an Arabidopsis mutant with constitutive defense whose size is roughly inversely proportional to SA levels. We found that, while mutations in CCA1 and LHY did not affect acd6-1 size [35] , the lux-1 mutation significantly suppressed acd6-1 dwarfism (Fig. 1a, b ). Compared with acd6-1 , acd6-1lux-1 also displayed decreased cell death, SA accumulation, expression of the defense marker gene PR1 , and resistance to the virulent P . syringae pv. maculicola ES4326 strain DG3 ( Pma DG3) (Fig. 1c–f ). The Col-0 and lux-1 plants appeared largely similar in their morphology except that lux-1 had slightly longer petioles. These results suggest a role of LUX in regulating SA-mediated defense. Fig. 1 The lux-1 mutation suppresses salicylic acid (SA)-mediated defense. a Phenotypes of 25-day-old plants. b Average size of 25-day-old plants. Plants were measured for the largest distance between tips of two rosette leaves ( n = 20). c Cell death staining of the fifth to seventh leaves of plants. d SA quantification. Whole plants were collected at ZT1 or ZT13 for SA extraction followed by high-performance liquid chromatography measurement ( n = 4 from two independent experiments). e Expression of PR1 . Whole plants of each genotype were collected at ZT1 or ZT13 for RNA extraction followed by quantitative reverse transcriptase–PCR (qRT-PCR) analysis ( n = 3). f Bacterial growth. The fourth to sixth leaves of each genotype were infiltrated with PmaDG3 (OD = 0.0001) at ZT1 or ZT13 and assessed for bacterial counts at 3 dpi ( n = 6). g SA quantification with plants infected by PmaDG3 . The fourth to sixth leaves of each genotype were infiltrated with PmaDG3 (OD = 0.01) or the mock solution at ZT1 and collected at the indicated time points for SA analysis ( n = 2). Data represent mean ± SD in d , e , g and mean ± SEM for b , f . Statistical analysis was performed with one-way analysis of variance with post hoc Tukey honestly significant difference test. Different letters in b , d – g indicate significant difference among the samples at the same time point ( P < 0.05). These experiments were repeated three times with similar results Full size image To further confirm this role of LUX , we challenged Col-0 and lux-1 plants with PmaDG3 and collected the infected leaves in a time course for SA quantification (Fig. 1g ). We found that there was a significant reduction in SA levels 16 and 20 h post infection (hpi) in lux-1 , as compared to Col-0. Thus these data support a role of LUX in regulating acute SA accumulation in local tissue upon P . syringae infection. LUX regulates multiple layers of defense responses The SA regulatory role of LUX suggests that LUX is important for plant disease resistance. Consistent with this idea, we found that expression of LUX was induced by infection with P . syringae strains, the virulent PmaDG3 and the avirulent strain Pma avrRpm1 (Supplementary Fig. 1 ). To further establish a role of LUX in defense regulation, we grew plants in a chamber with 12 h light/12 h dark (LD) and 180 µmol m −2 s −1 light intensity for 25 days and spray-infected the plants with Pma DG3 at zeitgeber time 1 (ZT1; ZT1 is 1 h after lights on) or ZT13 (1 hour after lights off). Infected plants were kept in continuous light (LL; a free running condition) and assessed for disease symptoms and bacterial growth. The infected lux-1 leaves displayed more chlorosis than those of Col-0 but did not show increased bacterial growth 4 days post infection (dpi) (Supplementary Fig. 2a ). The increased chlorosis in lux-1 is consistent with the role of LUX as a repressor of leaf senescence [36] . High light intensity exacerbates the senescence phenotype in lux-1 , complicating plant defense responses. To better assess the role of LUX in defense regulation, we lowered the light intensity from 180 to 10 µmol m −2 s −1 photon flux density in LL during infection (Fig. 2a ). Under these conditions, Col-0 showed time-of-day-dependent defense, depending on the mode of P . syringae infections [35] . To sprayed Pma DG3, Col-0 was more susceptible at LL25 (subjective morning) than at LL37 (subjective evening) (Fig. 2b and ref. [35] ). Interestingly, while the two lux mutants showed greater bacterial growth and more chlorosis than Col-0 with both LL25 and LL37 infections, lux demonstrated higher sensitivity to Pma DG3 in the morning than at night (Fig. 2b ). To infiltrated Pma DG3, Col-0 was more susceptible at night than in the morning (Fig. 2c and refs. [35] , [37] , [38] ). Such time-dependent susceptibility was abolished in lux , which demonstrated similar Pma DG3 growth when infected at both LL25 and LL37 but more bacterial growth than Col-0 at LL25 (Fig. 2c ). Expressing the wild-type LUX gene translationally fused to the GFP reporter in lux-4 ( LUX-GFP ) [6] , [39] rescued lux- conferred Pma DG3 susceptibility with infection at both LL25 and LL37 (Fig. 2b, c ). Fig. 2 LUX regulates stomata aperture and defense signaling. a Light and time scheme used for some treatments. 25-day-old plants grown in LD were transferred to LL for 1 day followed by pathogen infection 25 or 37 h after onset of LL. The light intensity was lowered from 180 to 10 µmol m −2 s −1 photon flux density at 49 h LL or 61 h LL for plants infected at 25 h LL or 37 h LL, respectively. b Bacterial growth (left) and photographs (right) of plants sprayed with PmaDG3 (OD 600 = 0.1) at LL25 or LL37 ( n = 6). c Bacterial growth of plants infiltrated with PmaDG3 (OD 600 = 0.0001) at LL25 (white bars) or LL37 (black bars) ( n = 6). d Stomatal aperture measured at 1 hpi of PmaDG3 (OD 600 = 0.1) at LL25 or LL37 ( n = 80). e Systemic acquired resistance (SAR) assay ( n = 6). SAR was induced by the primary infection of Pma avrRpt2 (OD = 0.05). Bacterial growth (left) and disease symptom (right) was recorded with the secondary infection of Pma DG3 (OD = 0.0001) at 3 dpi in LD. f Seedling growth inhibition assay with 1 µM flg22. The fold difference was calculated as the ratio of water-treated root length/flg22-treated root length of each genotype. Data (left) represent the average of three independent experiments ( n = 4 per genotype/treatment in each experiment). Pictures of seedlings (right) were from one representative experiment. g Quantification (left) and images (right) of callose deposition with flg22 (1 µM) or Pma hrcC − (OD 600 = 0.1) treatment ( n = 6). Numbers of callose deposits were quantified using ImageJ (version 1.45). H 2 O treatment did not induce callose deposition (not shown). Data represent mean ± SEM. Except f , other experiments were repeated two times and similar results were obtained. Statistical analysis was performed with one-way analysis of variance with post hoc Tukey honestly significant difference test. Significant difference between Col-0 and other plants at the same time point and/or with the same treatment was indicated by different letters or by asterisks (one asterisk for P < 0.05, two for P < 0.01, and three for P < 0.001) Full size image Because sprayed Pma DG3 gains access to the interior of plant tissue via stomata, we examined whether LUX affects stomata-dependent defense. In LL, Col-0 and LUX-GFP plants showed circadian-regulated stomatal aperture, with stomata more open in the morning than at night (Fig. 2d and Supplementary Fig. 2b ). Consistent with them being arrhythmic, the lux mutants lost this temporal modulation of stomatal activity and kept stomata open at both LL25 and LL37. When being challenged with Pma DG3 in LL, Col-0 and LUX-GFP plants demonstrated a temporal stomatal response (Fig. 2d and Supplementary Fig. 2b ). At LL25, 1 h Pma DG3 incubation transiently induced stomatal closure in Col-0 and LUX-GFP plants. At LL37, the stomatal aperture of Col-0 and LUX-GFP plants did not change within 3 h of exposure to Pma DG3. In contrast to Col-0 and LUX-GFP , the lux mutations disrupted this temporal response of stomata to Pma DG3 challenge. At LL25, the stomatal aperture of lux incubated for 1 h with Pma DG3 was smaller than that of mock-treated lux but was still significantly larger than that of Pma DG3-infected Col-0. At LL37, stomata of lux responded strongly to Pma DG3, showing significantly smaller aperture at 1 hpi than those of lux at 1 hpi at LL25. Open stomata observed in the lux mutants at LL37 could allow Pma DG3 to enter and thereby infect plant tissue, making the lux plants more susceptible than Col-0. The higher sensitivity of lux stomata to acute Pma DG3 infection at night than in the morning explains why the lux mutants showed more resistance at night than in the morning. Together, our data suggest that LUX regulates temporal defense in both stomata-dependent and stomata-independent pathways. We further tested whether LUX is involved in activating defense signaling. Recognition of a pathogen avirulence effector by its cognate resistance protein in the local infected tissue often results in enhanced and durable resistance in distal uninfected regions, termed systemic acquired resistance (SAR). To test whether LUX affects SAR, we infiltrated at ZT1 the fourth to sixth leaves of Col-0, lux-1 , and lux-4 plants with Pma avrRpt2 to activate SAR or with a mock solution as a control. At ZT1 2 dpi, we challenged the plants with a secondary infection of PmaDG3 . As expected, SAR-activated Col-0 plants showed more resistance to PmaDG3 , compared with non-SAR-activated Col-0 (Fig. 2e ). In contrast, no difference was observed in the lux mutants with the initial mock or Pma avrRpt2 treatment. These results suggest that LUX is necessary for SAR activation. To test whether LUX affects basal defense, we used flg22, a 22 aa peptide from the conserved region of the flagellin protein of P . syringae , to elicit basal immunity, also known as pathogen-associated molecular pattern-triggered immunity (PTI) [40] . We assayed two physiological changes associated with flg22-PTI, seedling growth inhibition and callose deposition [40] , [41] . We found that the lux-1 mutant was less sensitive than Col-0 in flg22-induced seedling growth inhibition and callose deposition (Fig. 2f, g ). We further challenged plants with another basal defense inducer, the Pma hrcC − strain that lacks the type III secretion system to deliver effectors to plant cells [20] . We found that Pma hrcC − induced significantly fewer callose deposits in lux-1 than in Col-0 (Fig. 2g ). Together, these data suggest that LUX contributes to basal defense in Arabidopsis. A role of LUX in regulating SA- and JA-mediated defense To elucidate how LUX is mechanistically linked to plant defense, we performed RNA-seq analysis. We generated transcriptome profiles of Col-0, lux-1 , acd6-1 , and acd6-1lux-1 at both ZT1 and ZT13 with the goal of identifying potential LUX target genes. After removing low-quality reads, an average of 79.8% of filtered reads were mapped to the genome sequence of Arabidopsis (Supplementary Fig. 3a ). Correlation dendrogram analysis indicated that all biological replicates of each sample clustered together. Expression profiles of the samples separated into two major groups based on acd6-1 or Col-0 background (Supplementary Fig. 3b ). In each group, the expression profile further clustered by time followed by the LUX genotype. These observations suggest that defense activation by acd6-1 influences the global transcriptomic profile more profoundly than either time of day or the circadian clock gene LUX . To identify LUX -affected genes, we compared four groups: (a) Col-0 vs. lux-1 at ZT1; (b) Col-0 vs. lux-1 at ZT13; (c) acd6-1 vs. acd6-1lux-1 at ZT1; and (d) acd6-1 vs. acd6-1lux-1 at ZT13. 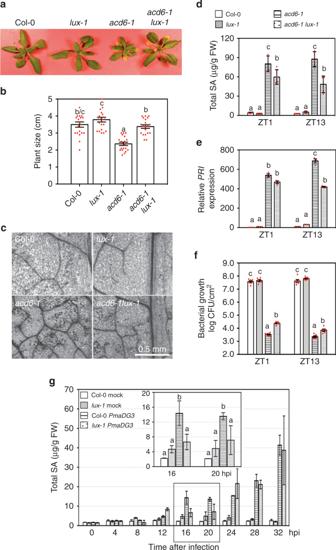Fig. 1 Thelux-1mutation suppresses salicylic acid (SA)-mediated defense.aPhenotypes of 25-day-old plants.bAverage size of 25-day-old plants. Plants were measured for the largest distance between tips of two rosette leaves (n= 20).cCell death staining of the fifth to seventh leaves of plants.dSA quantification. Whole plants were collected at ZT1 or ZT13 for SA extraction followed by high-performance liquid chromatography measurement (n= 4 from two independent experiments).eExpression ofPR1. Whole plants of each genotype were collected at ZT1 or ZT13 for RNA extraction followed by quantitative reverse transcriptase–PCR (qRT-PCR) analysis (n= 3).fBacterial growth. The fourth to sixth leaves of each genotype were infiltrated withPmaDG3(OD = 0.0001) at ZT1 or ZT13 and assessed for bacterial counts at 3 dpi (n= 6).gSA quantification with plants infected byPmaDG3. The fourth to sixth leaves of each genotype were infiltrated withPmaDG3(OD = 0.01) or the mock solution at ZT1 and collected at the indicated time points for SA analysis (n= 2). Data represent mean ± SD ind,e,gand mean ± SEM forb,f. Statistical analysis was performed with one-way analysis of variance with post hoc Tukey honestly significant difference test. Different letters inb,d–gindicate significant difference among the samples at the same time point (P< 0.05). These experiments were repeated three times with similar results Table 1 shows that the number of genes affected by lux-1 was generally higher in the day (groups a and c) than at night (groups b and d). There were more downregulated genes in the morning (groups a and c) and more upregulated genes in the evening (groups b and d). Under non-defense activation conditions (the Col-0 background; groups a and b), there were 790 genes differentially affected by lux-1 at ZT1 and ZT13, less than the number of genes (1180) affected under defense activation conditions (the acd6-1 background; groups c and d) (Supplementary Fig. 4a, b ). A total of 1618 genes was found to be differentially affected by lux-1 in at least one of the comparison groups (Table 1 and Supplementary Fig. 4c ). Gene Ontology (GO) analysis of the LUX- affected genes revealed an enrichment of genes responding to abiotic and biotic stimuli in each comparison group and in all four groups combined, compared with the genome-wide gene expression profile (Table 1 ). Table 1 Biotic and abiotic stress-related genes are preferentially regulated by LUX Full size table Cluster analysis of the 1618 LUX -affected genes revealed three major groups (Fig. 3a ). Expression of many genes in group II was relatively low in all four genotypes, compared with expression in groups I and III. Some genes in group II showed greater expression in lux-1 , consistent with the known role of LUX as a transcriptional repressor. Most genes in group I were highly induced in acd6-1 . Expression of most group I and III genes was suppressed by lux-1 , especially at ZT1 and/or in the acd6-1 background, suggesting that LUX can also positively affect gene expression via direct or indirect means. GO analysis revealed that groups I and III were more enriched than group II in genes responding to abiotic and biotic stimuli (Fig. 3a ). Among the stress-related genes, expression of several PTI and SA genes was downregulated in lux-1 . Examples of these genes include PTI signaling genes, such as MPK3 , WRKY22 , and WRKY33 , and SA-associated genes, such as the major SA biosynthesis gene ICS1 , the SA regulatory genes EDS1 , PAD4 , and PBS3/WIN3/GDG12 , the SA receptors NPR1 and NPR3 , and the SA marker gene PR1 . Quantitative reverse transcriptase–PCR (qRT-PCR) analysis confirmed expression of some of these genes (Supplementary Fig. 5 ). Together, these data support a positive role of LUX in regulating both PTI- and SA-mediated defense. We also noticed altered expression of a number of genes related to JA signaling in lux-1 , including several JA regulatory genes (e.g., JAZ1 , JAZ5 , JAZ7 , and JAZ8 ) and JA marker genes (e.g., PDF1;2 , VSP1 , and VSP2 ) (Fig. 3a and Supplementary Fig. 5 ). These observations support a role of LUX in regulating JA signaling. Fig. 3 Elucidation of LUX target genes via RNA-seq and chromatin immunoprecipitation (ChIP) experiments. a Heatmap analysis of 1618 LUX -affected genes. Relative RPKM values of LUX -affected genes were used in the cluster analysis, using the heatmap.2() function in the R package gplots. b – f ChIP experiments detect in vivo association of LUX with the promoters of clock and defense genes. ChIP assays were performed with LUX-GFP plants or Col-0 expressing CAB2:LUC as the negative control [39] . Anti-GFP antibodies were used for IP, using mock treatment as a control. Each amplicon from a specific primer pair at the indicated position (relative to the transcription start site) in each gene promoter was quantified after normalization with the internal control ( UBQ ). Asterisks indicate the predicted LUX-binding site within the 1500-bp promoter region upstream of the transcription start site of each gene. Data represent mean ( n = 2) ± SD. This experiment was repeated four times for EDS1 and JAZ5 and two times for LNK1 , LNK2 , and CDF1 and similar results were obtained Full size image The LUX protein has been shown to bind to the LBS motif in some clock gene promoters [7] , [12] . In order to uncover additional direct LUX targets, we identified the LBS motifs in both sense and antisense directions within 1500 bp upstream of the transcription start site of selected LUX-affected defense genes (Supplementary Table 1 ). We conducted chromatin immunoprecipitation (ChIP) with these gene promoters, using the LUX-GFP plants and Col-0 plants expressing the luciferase reporter driven by the CAB2 gene promoter ( CAB2:LUC ) as a control [39] . Among the defense gene promoters tested, we detected LUX binding to the LBS motifs in the promoters of the SA regulator EDS1 and the JA regulator JAZ5 (Fig. 3b, c ). The lack of LUX binding to the regions distal to the LBS motif in these gene promoters validated the specificity of our ChIP experiments. Thus LUX may act, at least in part, through EDS1 and JAZ5 in regulating SA and JA signaling, respectively. To further test the role of LUX in JA signaling, we treated lux-1 and Col-0 seedlings with methyl jasmonate (MJ) and found that lux-1 was less sensitive to MJ than Col-0 in the root growth assay (Fig. 4a ). Under PmaDG3 challenge, the lux mutant accumulated much higher levels of JAZ5 , MYC2 , VSP1 , and VSP2 transcripts, supporting a repressor role of LUX in regulating JA-related gene expression (Fig. 4b ). Interestingly, the expression of EDS1 was lower in lux-1 upon PmaDG3 infection, suggesting the possibility that LUX acts as a transcriptional activator for EDS1 . Fig. 4 Mutations in LUX and EDS1 affect jasmonic acid response and signaling. a Root length inhibition with methyl jasmonate (MJ) treatment. The fold difference of seedling root length (left) was calculated as the ratio of seedling root length with water treatment/seedling root length with 10 µM MJ treatment. The MJ-insensitive mutant jar1-1 [68] was used as a negative control. Data (left) represent mean ± SEM of three independent experiments ( n = 6 seedlings per genotype/treatment in each experiment). Photographs of the seedlings (right) are from one representative experiment. b Quantitative reverse transcriptase–PCR (qRT-PCR) analysis of gene expression affected by lux-1 upon Pma DG3 infection ( n = 2). c qRT-PCR analysis of gene expression affected by eds1-2 upon Pma DG3 infection ( n = 2). d Disease rating of Botrytis -infected leaves. Plants were sprayed with Botrytis (2 × 10 5 spores/ml) 25 or 37 h after onset of LL and the fourth to sixth leaves of each genotype were scored for disease symptoms 4 dpi (121 or 133 h after onset of LL) using the following rating scale: 1 = no lesion or small rare lesions; 2 = lesions on 10–30% of a leaf; 3 = lesions on 30–50% of a leaf; 4 = lesions on 50–70% of a leaf; 5 = lesions on >70% of a leaf. Data (left) represent mean ± SEM of three independent experiments ( n = 30 leaves per genotype in each experiment). Statistical analysis was performed with one-way analysis of variance with post hoc Tukey honestly significant difference test. For a – c , different letters indicate significant difference among the samples at the same time point. For d , asterisks indicate significant difference in the same disease scale category between Col-0 and other genotypes. The experiments in b , c were repeated two times and similar results were obtained Full size image EDS1 was shown previously to function in both SA-dependent and SA-independent pathways [27] , [32] , [42] . We found that, like lux-1 , eds1-2 was less sensitive than Col-0 to MJ treatment in the root growth assay (Fig. 4a ). Expression of MYC2 , JAZ5 , VSP1 , and VSP2 was more induced in eds1-2 than in Col-0 upon PmaDG3 infection (Fig. 4c ). These results indicate a role of EDS1 in negatively regulating JA gene expression. JA signaling is known to be important for plant defense against necrotrophic pathogens, such as Botrytis cinerea . To test whether LUX regulates broad-spectrum disease resistance, we spray-infected whole Col-0 and LUX misexpressing plants with Botrytis at LL25 or LL37. We found that the lux mutants showed more severe necrotic lesions on the leaves than Col-0 and LUX-GFP plants with both infections (Fig. 4d ). Similarly, the loss-of-function mutant of the LUX- interactor gene ELF3 , elf3-7 , also showed enhanced susceptibility to Botrytis at both times, consistent with the previous result of the Botrytis assay with detached leaves [43] . Thus both LUX and its interacting protein ELF3 are important for plant resistance to the fungal pathogen Botrytis . Interestingly, unlike the lux mutants, eds1-2 was not compromised in its response to Botrytis infection (Fig. 4d ). Together, our data suggest that LUX affects both SA- and/or JA-mediated signaling, ultimately influencing defense outcome in Arabidopsis. An expanded role of LUX in regulating clock TTFLs and output To find LUX -affected genes that also oscillate in expression throughout the day, the web-based tool Phaser [44] , [45] was used to analyze gene expression in LD and LL, using publicly available microarray data [46] , [47] . Of the 1618 LUX- affected transcripts, 26.7% cycled under LD and 26.3% cycled under LL. When we analyzed the entire Arabidopsis transcriptome, we found that 18.9% cycled in LD and 17.8% in LL. This observation of enrichment of cycling transcripts in the set of LUX-affected transcripts suggests that LUX preferentially regulates the expression of cycling genes, consistent with LUX being a core clock regulator. Consistent with LUX being a transcription repressor, expression of many clock-regulated genes was higher in lux-1 . These genes include core clock genes (e.g., BOA , ELF4 , GI , LNK1 , LNK2 , PRR5 , PRR7 , PRR9 , and LUX itself) and clock output genes that regulate plant growth ( PIF4 ) [39] , flowering time control ( CDF1 , CO , FLC , and FT ) [48] , [49] , and cold response ( CBF1 , CBF2 , and CBF3 ) [50] . These genes are expressed with peaks at multiple and distinct times of day [9] , suggesting that the evening clock gene LUX has a profound influence on global gene expression at different times of day. It is important to note that, although known as an arrhythmic mutant in LL, lux-1 shows robust driven rhythms in gene expression in LD that, at least for the CAB2:LUC or GRP7:LUC reporters, is indistinguishable from that in WT seedlings [6] . We confirmed this rhythmic gene expression in lux-1 in LD by qRT-PCR (Supplementary Fig. 6 ). We found that PRR9 , PRR7 , PRR5 , and LUX showed distinct expression peaks in Col-0, which are similar to those in lux-1 . Expression of these genes was higher in lux-1 than in Col-0 at each time point tested, consistent with LUX-repressing expression of these genes. In addition, we previously showed that acd6-1 does not affect clock activity [35] . Therefore, we believe that the altered expression of cycling genes affected by lux-1 in the RNA-seq analysis is unlikely due to altered circadian phase among Col-0, lux-1 , acd6-1 , and acd6-1lux-1 . Nevertheless, because there were only two time points (ZT1 and ZT13) used in the RNA-seq analysis, we may have missed some cycling genes that are affected by LUX at other times of day. LUX was shown to bind to the LBS motifs in the promoters of GI , LNK1 , PRR7 , PRR9 , and LUX itself [7] , [12] , [51] . We confirmed the binding of LUX to these gene promoters by ChIP experiments (Supplementary Table 1 ). Further ChIP experiments with selected LUX -affected clock genes revealed additional LUX-binding targets, including a second LBS in the LNK1 promoter (Fig. 3d , the LNK1 position and ref. [51] ) and sites in the promoters of LNK2 (a homolog of LNK1 [52] , [53] ) and CDF1 (a flowering repressor gene [48] ) (Fig. 3e, f ). Overall, our data expand the set of LUX direct targets that participate in clock TTFLs and output pathways. Reciprocal regulation of clock activity by JA signaling Data from this report and previous studies [16] , [36] , [37] have established a circadian control of JA signaling. Whether JA signaling affects clock activity has not been reported previously. To test this possibility, we first examined the expression of several clock genes in Col-0 seedlings treated with 100 µM MJ in LL and found a suppression of LUX , CCA1 , and GRP7 transcripts within a 24-h treatment (Supplementary Fig. 7 ). To further test whether MJ affects clock activity, we monitored luciferase reporter activity driven by the CCA1 promoter ( CCA1:LUC ) in Col-0 seedlings. MJ inhibited CCA1:LUC /Col-0 seedling growth in a dosage-dependent manner (Supplementary Fig. 8a ). After normalization of the amplitude to seedling leaf area, we found that MJ dampened the amplitude of CCA1:LUC , regardless whether MJ was applied at LL25 or LL37 (Supplementary Fig. 9a ). Neither the period nor the phase of CCA1:LUC /Col-0 were affected (Supplementary Fig. 9c, d ). We further introduced the CCA1:LUC reporter into the coronatine insensitive 1-17 ( coi1-17 ) mutant that has an impaired JA receptor [33] , [34] , [54] . MJ did not affect seedling growth (Supplementary Fig. 8a ) or the amplitude, period, or phase of CCA1:LUC rhythmic expression in coi1-17 (Supplementary Fig. 9e–h ). Thus MJ-induced amplitude dampening of the circadian clock requires an intact JA receptor. MJ suppression of plant growth makes it difficult to distinguish the direct effect of MJ on clock activity from secondary effects due to its growth inhibition. To further test whether JA signaling could reciprocally affect clock activity, we used JA-isoleucine (JA-Ile), a major bioactive JA derivative that binds to COI1 to activate JA signaling [55] . JA-Ile did not cause seedling growth inhibition (Supplementary Fig. 8b ), suggesting that these two chemicals act differently to regulate plant growth. Similar to MJ, JA-Ile induced drastic amplitude dampening in both CCA1:LUC and GRP7:LUC reporters in Col-0 in a dosage-dependent manner (Fig. 5a, b, i, j ). The period of both reporters in Col-0 was significantly lengthened, albeit by <1 h, with 100 µM JA-Ile treatment (Fig. 5c, k ). We did not observe phase change of the two reporters with JA-Ile treatment (Fig. 5d, l ). In addition, JA-Ile did not induce changes of amplitude, period, and phase of CCA1:LUC in coi1-17 (Fig. 5e–h ). Thus these data support responsiveness of the circadian clock to JA signaling and, in whole, demonstrate reciprocal regulation between the circadian clock and JA signaling. Fig. 5 Activation of jasmonic acid (JA) signaling reciprocally affects clock activity. Five-day-old seedlings entrained in LD were transferred to LL for 1 day and were treated with JA-isoleucine (JA-Ile). Luminescence was recorded at 1-h intervals for 5 days and analyzed for amplitude, period, and phase with the R package MetaCycle. a – d Expression of CCA1:LUC in Col-0 treated with JA-Ile 25 h (top) or 37 h (bottom) after onset of LL. e – h Expression of CCA1:LUC in coi1-17 treated with JA-Ile 25 h (top) or 37 h (bottom) after onset of LL. i – l Expression of GRP7:LUC in Col-0 treated with JA-Ile 25 h (top) or 37 h (bottom) after onset of LL. a , e , i Luminescence traces. RLU relative luminescence units. The color indicates JA-Ile concentration, black for 0 μM, magenta for 10 μM, and gray for 100 μM. b , f , j Amplitude. c , g , k Period. d , h , l Phase shift. Data represent mean (±SEM) of three independent experiments ( n = 8 or 12 for each experiment). Statistical analysis was performed by one-way analysis of variance post hoc Tukey honestly significant difference test. Different letters indicate significant difference among the samples ( P < 0.05) Full size image Recent studies have established the role of the circadian clock in regulating plant innate immunity. However, the mechanisms underlying this role of the circadian clock are still not well understood. Here we illuminate that the core clock component LUX affects temporal behavior of the stomata to pose physical barrier and modulates key defense signaling mediated by SA and JA, leading to broad-spectrum disease resistance to pathogens and pests. Our data also identify additional LUX targets participating in clock TTFLs and output pathways. We further find that activation of JA signaling can feed back to influence clock activity. Plants are known to employ different mechanisms to fight against pathogens and pests with different lifestyles at different times of day. For infiltrated P . syringae , plants with a normal circadian clock show higher susceptibility at night than in the morning (Fig. 2c and refs. [35] , [37] , [38] ). For epiphytic bacterial pathogens, such as spray-infected P . syringae , plants show higher susceptibility in the morning than at night. Because epiphytic bacteria need to pass through stomata to gain access to the interior of plant tissue and the infiltrated bacteria bypass this physical barrier, the differential resistance of plants to pathogens with different infection modes suggests that stomata-independent defense is strong during the day while stomata-dependent defense is dominant at night [35] . Our data show that the lux mutants lose the temporal defense demonstrated by Col-0 in response to both infiltrated and sprayed P . syringae (Fig. 2b, c ), suggesting a role of LUX-mediated circadian control of stomata-dependent and stomata-independent defense. The lux mutants, like Col-0 plants, showed higher resistance to sprayed P . syringae in the subjective evening than in the subjective morning, although at both infection time points, the lux mutants were more susceptible than Col-0 (Fig. 2b ). These observations appear to suggest that the circadian clock does not contribute to defense against epiphytic bacteria. However, our further analysis of the change of stomatal aperture led us to reject this notion. We found that, in LL without P . syringae infection, the lux mutant lost temporal oscillation of stomatal aperture exhibited by Col-0 (Fig. 2d and Supplementary Fig. 2b ). In the presence of P . syringae , stomata of Col-0 were highly sensitive for aperture reduction in the morning but showed no response at night due to the closure of stomata. In contrast, the lux mutants lost this temporal gating of the response to acute P . syringae infection, showing stomatal aperture reduction both in the morning and at night and being even more sensitive to the bacteria at night. Therefore, our data support that the lux mutations disrupt the circadian clock and subsequently abolish this temporal variation in stomata-dependent defense. Because the lux mutations do not completely abolish P . syringae- induced stomatal aperture reduction in the morning, LUX likely only partially affects stomata-dependent defense, and additional factors also contribute to this defense. In contrast, plants use different defense mechanisms in response to challenge by the necrotrophic fungal pathogen Botrytis and are less dependent on stomata-dependent defense. Accordingly, the lux mutants infected with Botrytis in the subjective evening are not more resistant than those infected in the subjective morning (Fig. 4d ). In addition to using physical barriers like stomata to exclude pathogens, plants can mount defense through activating cellular signaling pathways. SA and JA are important defense signaling molecules. SA is generally considered to be important for defense against biotrophic pathogens, whereas JA promotes resistance to necrotrophic pathogens and insects [56] , [57] , [58] . Crosstalk between SA and JA determines the balance of plant defense against pathogens and pests with different lifestyles. However, how the circadian clock affects SA- and JA-mediated defense is complex and not completely understood. We report here a role of LUX in regulating SA and JA signaling. The lux-1 mutation suppresses high SA accumulation in acd6-1 and results in reduced SA levels during acute defense responses in the presence of P . syringae (Fig. 1 ). RNA-seq analysis reveals that expression of many SA-related genes are affected by lux-1 . Our detection of a direct binding of LUX to the promoter of EDS1 , a major SA regulator involved in the SA signal amplification loop [27] , [42] , suggests that this SA regulatory role of LUX could be, at least in part, mediated through EDS1 . The lux-1 mutant also demonstrates lower sensitivity to MJ treatment and altered JA gene expression relative to Col-0 (Figs. 3a and 4 ). LUX was previously shown to bind to the promoter of MYC2 , a JA transcription factor [36] . We report here a direct binding of LUX to the promoter of the JA signaling repressor JAZ5 . Interestingly, our data show that eds1-2 is less sensitive to MJ and has increased expression of JA-related genes upon P . syringae infection. Thus EDS1 is also involved in JA signaling. This role of EDS1 could be due to EDS1 -mediated crosstalk between SA and JA signaling. Alternatively, it is also possible that EDS1 exerts direct influence on JA signaling in an SA-independent manner [27] , [42] . Indeed, a recent study showed that two EDS1 interactors, PHYTOALEXIN DEFICIENT 4 (PAD4) and SENESCENCE-ASSOCIATED GENE 101 [59] , [60] , interacted with MYC2 in a transient assay [61] . EDS1–PAD4 binding could compete for PAD4–MYC2 interaction and therefore affect JA signaling. Together, these data indicate that LUX could gate JA signaling by directly controlling multiple JA signaling components. Our study revealed the role of LUX in mediating SA and JA signaling, thus providing a mechanistic explanation for the crosstalk between the circadian clock and defense. Consistent with this role of LUX , loss of function in LUX confers compromised resistance to a broad spectrum of pathogens and pests with different lifestyles, including the herbivorous insect Trichoplusia ni (cabbage looper), the biotrophic bacterial pathogen P . syringae , and the necrotrophic fungal pathogen Botrytis (Figs. 2 and 4d ) [16] . In addition to LUX, other clock genes may affect plant defense through SA and JA signaling. Among previously reported clock genes with roles in defense regulation, CCA1 and LHY act largely in an SA-independent manner [35] . Like lux , arrhythmia caused by overexpression of CCA1 blocked resistance to cabbage loopers [35] , [62] . Whether CCA1 acts similarly as LUX in affecting JA signaling and subsequently insect resistance remains to be determined. Another clock gene, CCA1 HIKING EXPEDITION ( CHE ), encodes a protein that binds to the promoter of the major SA synthase gene ICS1 [17] . CHE was shown to be important for diurnal SA biosynthesis both in the absence of pathogens and during P . syringae -induced SAR. Whether CHE gates local acute SA biosynthesis upon pathogen infection is currently unknown. The clock protein TIC was shown to regulate JA signaling through a direct interaction with the JA transcription factor MYC2 [37] . It is not known, however, whether TIC acts through the JA pathway to modulate the disease outcome of plants in the presence of pathogens and pests. Thus it would be pertinent to reveal the molecular mechanism underlying the function of clock genes in their control of plant defense. Because SA and JA are important defense signaling molecules, multiple regulatory inputs to SA and JA signaling from the circadian clock allow plants to continuously monitor the change of these signaling pathways to ensure proper growth, development, and response to external stimuli. Both SA and JA levels as well as expression of some genes involved in SA and JA biosynthesis and signaling oscillate under non-challenged conditions [1] . The cycling expression of most clock genes necessitates the use of clock genes expressed at distinct circadian phases in order to provide inputs to SA and JA signaling at multiple times of day. The circadian clock is also likely important to gate SA and JA signaling under acute stress conditions. While establishing regulation by LUX of plant innate immunity, we realize the complexity of host–pathogen interactions, the outcome of which is likely influenced by multiple other factors in addition to the circadian clock. We observed enhanced disease susceptibility of the lux mutants in LL with a light intensity of 10 µmol m −2 s −1 photon flux but not with 180 µmol m −2 s −1 photon flux. These results suggest that the defense role of the circadian clock is conditional and influenced by light. The EC, consisting of LUX-ELF3-ELF4, is known to regulate light signaling through affecting expression of many photosynthesis genes and light responsive genes [63] . Thus mutations in LUX or other EC genes could make plants particularly sensitive to light, complicating pathogen response. Although 10 µmol m −2 s −1 photon flux is a relatively low light intensity, compared with the conditions typically used for plant growth in the laboratory, such light intensities are encountered in deeply shaded conditions and every day during twilight after dawn and prior to dusk. In addition, both LL and DD have been routinely used as free running conditions to test clock activities in plants, animals, and fungi in laboratory conditions. Therefore, our use of this low light regime is physiologically relevant. In addition to light intensity, other factors, such as light duration and temperature, contribute to LUX-regulated processes. For instance, the early flowering phenotype conferred by the lux mutations is more evident in 8 h L/16 h D than in 16 h L/8 h D [6] . The transcriptional targets of LUX (and its interactor ELF3) are temperature dependent, suggesting a temperature input to EC function [63] , [64] . Together, these observations suggest the complexity of circadian regulation of biological processes, which can be further compounded by additional factors that modulate the process either directly or indirectly via an effect on the circadian clock. In addition to defense control, our data support the importance of LUX in maintaining clock function, likely through a direct control of expression of core clock TTFL genes and genes in output pathways. A recent ChIP-seq study reported >800 LBSs in Arabidopsis [63] , supporting this notion. Our bioinformatics analysis followed by ChIP experiments revealed additional new targets of LUX, including EDS1 , JAZ5 , LNK2 , and a second LBS motif in the LNK1 promoter. We also detected LUX binding to the CDF1 promoter, which was shown as one of the LUX targets in the ChIP-seq experiment but had not been independently verified [63] . LUX likely acts as a transcriptional repressor to affect the expression of many target genes. It is also possible that LUX positively regulates gene expression (Figs. 3 and 4b ). This gene activation role of LUX could be indirect and reflect LUX’s repression of another repressor important for the regulation of gene transcription. Alternatively, the LUX protein might activate target gene expression through recruitment to promoters, including that of EDS1 , as part of as yet undescribed transcriptional activation complex. Together, the detection of widespread targets of LUX in Arabidopsis genome supports the importance of LUX in regulating the circadian clock and other biological processes. While the circadian clock regulates multiple output pathways, including plant development and responses to environmental stimuli, many of these output pathways are known to reciprocally regulate clock activity [1] . Such reciprocal regulation likely represents a mechanism to integrate environmental cues with proper growth and development. This report and those from other researchers establish a reciprocal regulation of the circadian clock and defense signaling mediated by SA and JA. SA was shown to delay the phase and dampen the amplitude of some clock reporters [65] . However, SA does not affect clock period [35] , [53] , [65] , [66] . We show here that JA-Ile dampens the amplitude and lengthens period of two clock reporters in wild-type Col-0. These observations were largely corroborated by those obtained with an JA-Ile analog, MJ. However, we also observed differences in the change of period and seedling growth with the two chemicals, suggesting that they have overlapping yet also distinct function in signal activation in plants. Together, this reciprocal regulation of the circadian clock by SA and JA signaling provides another layer of monitoring of these defense pathways, which can be reset by their own feedback modulation of circadian clock function. That LUX regulates JA signaling and that LUX expression is also influenced by JA clearly suggest LUX is a key, although not necessarily the sole, node in mediating crosstalk between the circadian clock and defense signaling involving JA. A better understanding of the role of the circadian clock in regulating plant growth, development, and responses to abiotic and biotic stresses in plants would tremendously advance our knowledge of basic science, as well as offer potential applications to improve crop yield and disease resistance. Misexpression of several core clock genes has been shown to compromise plant immunity to pathogens and pests. However, it remains unclear how individual clock genes work together to integrate endogenous and exogenous cues to regulate the circadian clock and defense. We demonstrate in this report that LUX directly targets important clock TTFL genes and output genes for transcriptional regulation and that LUX-mediated defense signaling also reciprocally regulates clock activity. Thus these data provide a mechanistic view of LUX function as a pivotal node connecting the circadian clock and defense. Future work revealing mechanisms of action of additional clock TTFL genes will shed more light on this exciting research field. Plant materials All plants used in this report are in the Col-0 background. Unless otherwise indicated, plants were grown in growth chambers with a light intensity at 180 µmol m −2 s −1 , 60% humidity, and 22 °C either in a 12 h light/12 h dark (LD) cycle. The lux-1 and elf3-7 mutants were kindly provided by Todd Michael (Craig Venter Institute); the lux-4 , lux-4 expressing LUX-GFP , and CAB2:LUC seeds were provided by Steve Kay (The University of Southern California); and the coi1-17 seed was provided by Barbara Kunkel (Washington University). The CCA1:LUC reporter was introduced into coi1-17 by crossing Col-0 expressing CCA1:LUC with coi1-17 , selfing, and identifying F2 lines homozygous for both the coi1-17 mutation and the CCA1:LUC reporter. The acd6-1lux-1 double mutant was generated by crossing two single mutants and selecting the homozygous double mutant in the F 2 generation, using derived cleaved amplified polymorphic sequence markers specific for each mutation. 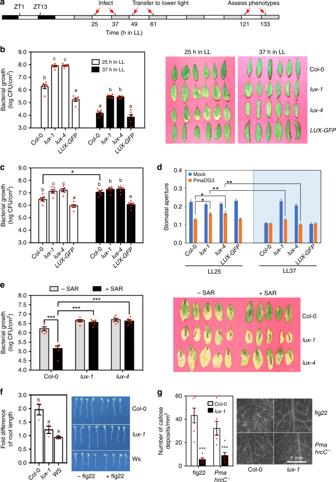Fig. 2 LUXregulates stomata aperture and defense signaling.aLight and time scheme used for some treatments. 25-day-old plants grown in LD were transferred to LL for 1 day followed by pathogen infection 25 or 37 h after onset of LL. The light intensity was lowered from 180 to 10 µmol m−2s−1photon flux density at 49 h LL or 61 h LL for plants infected at 25 h LL or 37 h LL, respectively.bBacterial growth (left) and photographs (right) of plants sprayed withPmaDG3(OD600= 0.1) at LL25 or LL37 (n= 6).cBacterial growth of plants infiltrated withPmaDG3(OD600= 0.0001) at LL25 (white bars) or LL37 (black bars) (n= 6).dStomatal aperture measured at 1 hpi ofPmaDG3(OD600= 0.1) at LL25 or LL37 (n= 80).eSystemic acquired resistance (SAR) assay (n= 6). SAR was induced by the primary infection ofPma avrRpt2(OD = 0.05). Bacterial growth (left) and disease symptom (right) was recorded with the secondary infection ofPmaDG3 (OD = 0.0001) at 3 dpi in LD.fSeedling growth inhibition assay with 1 µM flg22. The fold difference was calculated as the ratio of water-treated root length/flg22-treated root length of each genotype. Data (left) represent the average of three independent experiments (n= 4 per genotype/treatment in each experiment). Pictures of seedlings (right) were from one representative experiment.gQuantification (left) and images (right) of callose deposition with flg22 (1 µM) orPma hrcC−(OD600= 0.1) treatment (n= 6). Numbers of callose deposits were quantified using ImageJ (version 1.45). H2O treatment did not induce callose deposition (not shown). Data represent mean ± SEM. Exceptf, other experiments were repeated two times and similar results were obtained. Statistical analysis was performed with one-way analysis of variance with post hoc Tukey honestly significant difference test. Significant difference between Col-0 and other plants at the same time point and/or with the same treatment was indicated by different letters or by asterisks (one asterisk forP< 0.05, two forP< 0.01, and three forP< 0.001) Primers for mutant detections are listed in Supplementary Table 2 . Pathogen infection P. syringae pv. maculicola ES4326 strains DG3 ( Pma DG3), Pma avrRpm1 , Pma avrRpt2 , and Pma HrcC − were used in this report. Freshly cultured bacteria were resuspended in 10 mM MgSO 4 . Plants were infiltrated or evenly sprayed with a bacterial solution at the indicated concentration, time, and light condition. For SAR induction, the fourth to sixth leaves of 25-day-old plants grown in LD were infiltrated with Pma avrRpt2 (optical density (OD) = 0.05). The leaves with the primary infection were mostly dead (a hypersensitive response) at 2 dpi and were detached. The adjacent two to three leaves were further infiltrated with Pma DG3 (OD = 0.0001) and the bacterial growth was assessed at 3 days post the secondary infection. Because the hypersensitive response in Arabidopsis was reported to be light dependent [67] , both the primary and secondary infections were conducted in LD. B. cinerea strain BO5-10 was kindly provided by Tesfaye Mengiste (Purdue University). Twenty-five-day-old plants grown in LD were moved to LL for 1 day before being sprayed with Botrytis (2 × 10 5 spores/ml) 25 or 37 h after onset of LL. Plants were further transferred 24 hpi to low-light LL with a light intensity of 10 µmol m −2 s −1 . Disease symptoms of leaves at the fourth to sixth positions were rated at 4 dpi (121 or 133 h after onset of LL). The rating scale was as the follows: 1 = no lesion or small rare lesions; 2 = lesions on 10–30% of a leaf; 3 = lesions on 30–50% of a leaf; 4 = lesions on 50–70% of a leaf; 5 = lesions on >70% of a leaf. SA quantification Leaves from P . syringae -infected or mock-treated 25-day-old plants or non-infected whole plants were collected at the indicated times for SA extraction and measurement by a high-performance liquid chromatography instrument (Shimadzu LC-20AT). Cell death staining The fifth to seventh leaves of 25-day-old plants were stained with a trypan blue solution for cell death and photographed with a Leica IC80 HD camera connected to a Leica M80 stereomicroscope. RNA analyses Total RNA was extracted with TRIzol reagent (Invitrogen) according to the manufacturer’s instruction. Primers used in qRT-PCR are listed in Supplementary Table 2 . Stomatal aperture measurement Twenty-five-day-old plants grown in LD (180 µmol m −2 s −1 light intensity, 60% humidity, 22 °C, and 12 h light/12 h dark cycle) were moved to LL (10 µmol m −2 s −1 light intensity, other parameters remained the same) for 1 day. The fifth to seventh leaves of each genotype were taken at LL25 or LL37 and mounted onto scotch tape at the abaxial side. The top layer of a leaf was peeled off and the tape with the lower layer of the leaf was cut and mounted on a glass slide for observation with an inverted microscope. For P . syringae treatment, leaves were incubated with PmaDG3 (OD 600 = 0.1) or sterile water at LL25 or LL37. Leaves were processed as above for stomata imaging at 0, 1, and 3 hpi. Immediately after leaf processing, images of at least three random regions of each of the three or more leaves of each genotype per treatment were taken with a camera (Canon Digital Rebel xsi, Japan) connected to an inverted microscope (Olympus Model IMT-2). Each stoma was measured for the width and the length using ImageJ (version 1.45). Stomatal aperture was determined by the ratio between the width and the length of a stoma. At least 80 stomata were used for calculating the average stomatal aperture of each genotype per treatment. Seedling growth assay with flg22 or MJ treatment Seeds were surface-sterilized in a bell jar with bleach vapor generated by slowly adding 3 ml of concentrated HCl into 100 ml bleach. The jar was immediately sealed with a lid for 3 h in a fume hood. Sterilized seeds were plated on agar plates containing 1/2 MS media supplemented with 1% sucrose (pH 5.7). 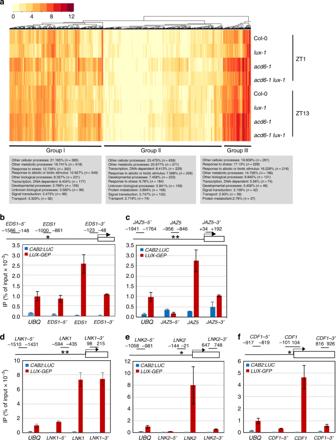Fig. 3 Elucidation ofLUXtarget genes via RNA-seq and chromatin immunoprecipitation (ChIP) experiments.aHeatmap analysis of 1618LUX-affected genes. Relative RPKM values ofLUX-affected genes were used in the cluster analysis, using the heatmap.2() function in the R package gplots.b–fChIP experiments detect in vivo association of LUX with the promoters of clock and defense genes. ChIP assays were performed withLUX-GFPplants or Col-0 expressingCAB2:LUCas the negative control39. Anti-GFP antibodies were used for IP, using mock treatment as a control. Each amplicon from a specific primer pair at the indicated position (relative to the transcription start site) in each gene promoter was quantified after normalization with the internal control (UBQ). Asterisks indicate the predicted LUX-binding site within the 1500-bp promoter region upstream of the transcription start site of each gene. Data represent mean (n= 2) ± SD. This experiment was repeated four times forEDS1andJAZ5and two times forLNK1,LNK2, andCDF1and similar results were obtained The plates were incubated at 4 °C for 2 days before being transferred to a tissue culture chamber in LD and 22 °C for 4 days. Seedlings were then transferred to a 24-well tissue culture plate with sterile water in the presence or absence of 1 µM flg22 or 10 µM MJ. At least four seedlings were used for each genotype per treatment. Root length of the seedlings was measured 4 days later. The Ws ecotype that does not have a functional flg22-receptor FLS2 [41] and the jar1-1 mutant that is insensitive to JA signaling [68] were used as a negative control for flg22 and MJ treatments, respectively. Callose staining Flg22- or Pma HrcC − - treated leaves were harvested at 24 hpi and boiled in alcoholic lactophenol (95% ethanol:lactophenol = 2:1) for 2 min followed by rinsing in 50% ethanol. Aniline blue solution (0.01% aniline blue in 150 mM KH 2 PO 4, pH 9.5) was used to stain the leaves for 1.5 h in dark. At least four leaves of each genotype were used in each treatment. Callose deposition was visualized with a Leica fluorescence stereomicroscope (M205 FA) and imaged with a CCD camera (Cool Snap HQ [2] , Photometrics, USA). Callose deposits were quantified using ImageJ (version 1.45). RNA-seq analysis Total RNA was extracted from 25-day-old Col-0, lux-1 , acd6-1 , or acd6-1lux-1 plants collected at ZT1 or ZT13 1 and 13 h after light onset, respectively. Triplicate biological samples were used for most genotypes at each time point, except acd6-1 and acd6-1lux-1 at ZT13, which had duplicate samples. In all, 0.5 μg RNA per replicate was used to generate cDNA libraries using the Illumina TruSeq RNA Sample Preparation Kit (catalog no. RS-122-2001). 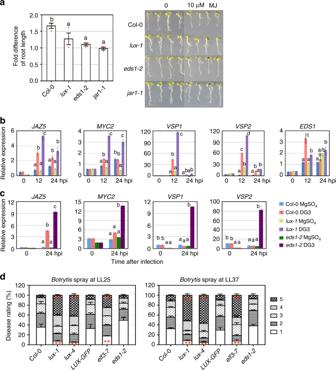Fig. 4 Mutations inLUXandEDS1affect jasmonic acid response and signaling.aRoot length inhibition with methyl jasmonate (MJ) treatment. The fold difference of seedling root length (left) was calculated as the ratio of seedling root length with water treatment/seedling root length with 10 µM MJ treatment. The MJ-insensitive mutantjar1-168was used as a negative control. Data (left) represent mean ± SEM of three independent experiments (n= 6 seedlings per genotype/treatment in each experiment). Photographs of the seedlings (right) are from one representative experiment.bQuantitative reverse transcriptase–PCR (qRT-PCR) analysis of gene expression affected bylux-1uponPmaDG3 infection (n= 2).cqRT-PCR analysis of gene expression affected byeds1-2uponPmaDG3 infection (n= 2).dDisease rating ofBotrytis-infected leaves. Plants were sprayed withBotrytis(2 × 105spores/ml) 25 or 37 h after onset of LL and the fourth to sixth leaves of each genotype were scored for disease symptoms 4 dpi (121 or 133 h after onset of LL) using the following rating scale: 1 = no lesion or small rare lesions; 2 = lesions on 10–30% of a leaf; 3 = lesions on 30–50% of a leaf; 4 = lesions on 50–70% of a leaf; 5 = lesions on >70% of a leaf. Data (left) represent mean ± SEM of three independent experiments (n= 30 leaves per genotype in each experiment). Statistical analysis was performed with one-way analysis of variance with post hoc Tukey honestly significant difference test. Fora–c, different letters indicate significant difference among the samples at the same time point. Ford, asterisks indicate significant difference in the same disease scale category between Col-0 and other genotypes. The experiments inb,cwere repeated two times and similar results were obtained 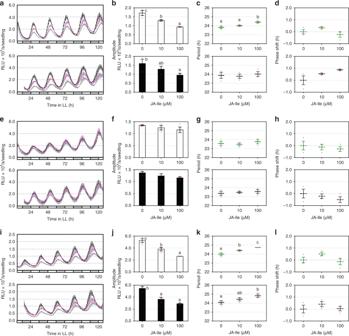Fig. 5 Activation of jasmonic acid (JA) signaling reciprocally affects clock activity. Five-day-old seedlings entrained in LD were transferred to LL for 1 day and were treated with JA-isoleucine (JA-Ile). Luminescence was recorded at 1-h intervals for 5 days and analyzed for amplitude, period, and phase with the R package MetaCycle.a–dExpression ofCCA1:LUCin Col-0 treated with JA-Ile 25 h (top) or 37 h (bottom) after onset of LL.e–hExpression ofCCA1:LUCincoi1-17treated with JA-Ile 25 h (top) or 37 h (bottom) after onset of LL.i–lExpression ofGRP7:LUCin Col-0 treated with JA-Ile 25 h (top) or 37 h (bottom) after onset of LL.a,e,iLuminescence traces. RLU relative luminescence units. The color indicates JA-Ile concentration, black for 0 μM, magenta for 10 μM, and gray for 100 μM.b,f,jAmplitude.c,g,kPeriod.d,h,lPhase shift. Data represent mean (±SEM) of three independent experiments (n= 8 or 12 for each experiment). Statistical analysis was performed by one-way analysis of variance post hoc Tukey honestly significant difference test. Different letters indicate significant difference among the samples (P< 0.05) The samples were multiplexed and sequenced using the Illumina HiSeq sequencing platform in Genomics Resources Core Facility at Weill Cornell Medical College. Sequencing was conducted with a standard run of 51 cycles and single reads [31] . At least 150 million reads per lane were obtained for sequencing. Differentially expressed genes in each comparison group were identified using the R package DESeq, using the default parameters [69] . The default false discovery rate of 0.1, which results in statistical significance with P values < 0.001, was used to define significant difference in the gene expression in each comparison group. For global gene expression profiling, the relative expression value (reads per kilobase of transcript per million mapped reads (RPKM)) of >0.3 was used as the cutoff to include genes for further analyses. Each RPKM value was corrected by adding the number one and then was log 2 -transformed for generating the correlation dendrogram with R function cor(). To show the number of overlapped genes affected among the comparison groups, Venn diagrams were generated with the R package VennDiagram. The GO annotations tool on the TAIR website was used to assign genes into functional groups. The whole-genome genes of Arabidopsis were also similarly analyzed to provide the reference number for GO annotation. Graphical representation of gene expression correlation was produced by the heatmap.2() function in the R package gplots. ChIP assays The ChIP experiments were conducted according to previous descriptions with modifications [7] , [70] . Fourteen-day-old wild-type CAB2:LUC or LUX-GFP ( lux-4 expressing LUX:LUX-GFP) seedlings grown on soil were harvested at ZT13. The seedlings were crosslinked by immersion into 30 ml of 1% formaldehyde solution at room temperature under vacuum for 20 min. Glycine (2 ml at 2 M concentration) was added to the seedlings for 5 min under vacuum to quench the crosslink reaction. The seedlings were then rinsed with water and stored at −80 °C for further use. The seedlings were ground in liquid nitrogen to a fine powder and extracted for DNA and protein with 30 ml of extraction buffer I (0.4% sucrose, 10 mM Tris-HCl pH8.0, 0.035% 2-mercaptoethanol, 1 mM phenylmethanesulfonylfluoride (PMSF), 5 mM benzamidine, 1× Roche protease inhibitors) in a 50 ml Falcon tube. The tube was incubated on ice for 15 min until the tissue was thawed. The solution was filtered through miracloth and centrifuged at 750 × g at 4 °C for 20 min. The pellet was resuspended in 1 ml of extraction buffer II (0.25 M sucrose, 10 mM Tris-HCl pH8.0, 10 mM MgCl 2 , 1% Triton X-100, 0.035% 2-mercaptoethanol, 1 mM PMSF, 5 mM benzamidine, 50 µM MG132, 1× Roche protease inhibitors) and centrifuged at 15600 g at 4 °C for 10 min. The remaining pellet was resuspended in 500 µl of extraction buffer III (1.7 M sucrose, 10 mM Tris-HCl pH8.0, 2 mM MgCl 2 , 0.15% Triton X-100, 0.035% 2-mercaptoethanol, 1 mM PMSF, 5 mM benzamidine, 50 µM MG132, 1× Roche protease inhibitors). The suspension was laid on the top of another 500 µl extraction buffer III in a 1.5 ml Eppendorf tube and centrifuged at 15,600 × g at 4 °C for 1 h. After removing the supernatant, the pellet was resuspended in 500 µl of nuclei lysis buffer (50 mM Tris-HCl pH8.0, 10 mM EDTA, 1% sodium dodecyl sulfate (SDS), 1 mM PMSF, 5 mM benzamidine, 50 µM MG132, 1× Roche protease inhibitors). The suspension was sonicated on ice (15 s pulse followed by 45 s resting, repeating 12 times) using a sonicator (Virsonic Cell Disruptor, Model 16-850) set at 30% power to shear genomic DNA to an average size of 500–1000 bp. The sonicated chromatin solution was centrifuged at 15,600 × g for 10 min at 4 °C and the supernatant was collected. This process was repeated one time and all supernatants containing the chromatin solution were combined. One hundred and fifty microliters of chromatin solution was then diluted in 1350 µl of ChIP dilution buffer (16.7 mM Tris-HCl pH8.0, 1.2 mM EDTA, 1.1% Triton X-100, 167 mM NaCl, 1 mM PMSF, 5 mM benzamidine, 50 µM MG132, 1× Roche protease inhibitors). Anti-GFP antibodies (IP) (Abcam, product code 290) or whole rabbit IgG (mock) (Jackson ImmunoResearch cat 011-000-003) coated onto Dynabeads Protein G (Invitrogen cat 100.04D) were used for IP. Diluted chromatin solution (700 µl/sample) was incubated with either IP- or mock-treated beads at 4 °C for 1.5 h. In the meantime, 70 µl diluted chromatin solution was kept aside as the input. After incubation, beads were washed at 4 °C with low salt buffer twice (20 mM Tris-HCl pH8.0, 150 mM NaCl, 0.2% SDS, 0.5% Triton X-100, 2 mM EDTA), high salt buffer once (20 mM Tris-HCl pH8.0, 500 mM NaCl, 0.2% SDS, 0.5% Triton X-100, 2 mM EDTA), and TE buffer twice. The beads were resuspended in 100 µl elution buffer (50 mM Tris pH8.0, 10 mM EDTA, 1% SDS) and incubated at 65 °C for 15 min followed by 30 s centrifugation at 376 × g to elute the immunocomplexes from the beads. The supernatant was transferred into a new 1.5 ml Eppendorf tube and was added with NaCl to the final concentration of 0.2 M and 1 µl of Proteinase K. All tubes (IP, mock, and input tubes for each sample) were incubated overnight at 65 °C to reverse crosslinking. Chromatin DNA was purified using a Qiagen QIAquick PCR Purification Kit and resuspended in 300 µl of water. ChIP DNAs were quantified by real-time qPCR with primers specific for the amplicons covering LBS motifs in gene promoters using a 3 µl aliquot from IP, mock, or input tubes for each sample. Fold enrichment for each promoter region in plants expressing LUX:LUX-GFP or CAB2:LUC was normalized with the input DNA and the internal control DNA (a fragment from the UBQ gene promoter) and was calculated using the following equation: 2 (Ct input − Ct IP) /2 (Ct input − Ct mock) . Primers for the ChIP experiments are listed in Supplementary Table 2 . Luciferase assay Seedlings expressing the CCA1 : LUC or GRP7 : LUC reporter were grown on 1/2 MS media with 1% sucrose in LD and at 22 °C for 5 days. Seedlings were transferred to 96-well plates containing 200 µl of 1/2 MS medium with 0.5% sucrose, 0.4% agar, and 0.25 mM D-luciferin for 1 day in LD followed by 1 day in LL with a light intensity of 180 µmol m −2 s −1 . Each well contained one seedling. Seedling treatments were conducted at LL25 or LL37 by adding 15 µl of each chemical (MJ (10 µM or 100 µM), JA-Ile (10 µM or 100 µM), or the mock solution (sterile water)) to each well. Immediately after the treatments, the plants were measured for luminescence with an Omega Luminescence Reader (BMG LABTECH, Inc.) in LL with 90 µmol m −2 s −1 photon flux density. LUC activity was measured at 1-h intervals for 5 days. Each microplate with seedlings was photographed after LUC recording. Leaf area of each seedling was measured using ImageJ (version 1.45). The amplitude, period, and phase were calculated with the R package MetaCycle [71] . Reporting summary Further information on research design is available in the Nature Research Reporting Summary linked to this article.